Susceptibility of memory consolidation during lapses in recall Memories that can be recalled several hours after learning may paradoxically become inaccessible for brief periods after their formation. This raises major questions about the function of these early memory lapses in the structure of memory consolidation. These questions are difficult to investigate because of the lack of information on the precise timing of lapses. However, the use of a single-trial conditioning paradigm in Lymnaea solves this problem. Here we use electrophysiological and behavioural experiments to reveal lapses in memory recall at 30 min and 2 h post conditioning. We show that only during these lapses is consolidation of long-term memory susceptible to interruption by external disturbance. These shared time points of memory lapse and susceptibility correspond to transitions between different phases of memory that have different molecular requirements. We propose that during periods of molecular transition memory recall is weakened, allowing novel sensory cues to block the consolidation of long-term memory. The structure of memory consolidation is of major current interest [1] , [2] , [3] . The main debate has concerned the status of reconsolidation, for instance, whether it is similar or different from consolidation. Reconsolidation refers to the process whereby long-term memories (LTM), following recall, enter a special labile state in which they become prone to change. However, lability is not confined to reconsolidation and there is considerable evidence that consolidation, the process that converts short-term memory (STM) to LTM, is also subject to plasticity in memory recall. Reports of temporary lapses in memory during consolidation are widespread in the literature and have been observed in many invertebrate [4] , [5] and vertebrate species [6] , [7] , [8] including humans [9] . But it is not clear what the functions of these lapses might be, especially when they occur at several time points. In this paper, we first investigate when after conditioning the lapses in memory occur and show how this maps onto transitions in memory consolidation as defined by their underlying molecular mechanisms. We then test the specific hypothesis that lapses in memory recall coincide with periods when consolidation of LTM is susceptible to disturbances from outside the memory network. We took advantage of the model molluscan system, Lymnaea , because associative conditioning of feeding using a single training trial leads to LTM that persists for up to 19 days. Single-trial training has the major advantage that it is possible to obtain data on the precise timing of subsequent electrical and molecular events that underlie the various phases of memory consolidation leading to LTM. We use the feeding behaviour of this animal because previous experiments revealed the detailed behavioural, electrophysiological and molecular mechanisms that underlie associative reward conditioning of feeding [10] , [11] , [12] , [13] , [14] , [15] , [16] . The development of a unique semi-intact preparation for in vitro conditioning [17] was particularly useful for recording electrical correlates of conditioning ‘in the dish’, and our knowledge of drug protocols that could block a variety of learning-induced molecular processes in the nervous system of Lymnaea [13] , [14] , [18] allowed us to study the roles of protein synthesis, RNA synthesis and protein kinases in consolidation. After in vitro and behavioural one-trial conditioning, we show lapses in memory at 30 min and 2 h but not 10 min, 1, 3 and 4 h. The lapse in memory expression at 30 min marks the transition from STM to intermediate-term memory (ITM). The 2 h lapse indicates that ITM has an early and a late phase, each with a different underlying specific molecular requirement. No lapses in memory occurred at the transition between late ITM and LTM that first occurred 4 h after training. We show that lapses in memory are critical time points of susceptibility to novel external stimuli. Disruptive external mechanical stimuli delivered at these time points, but not at others, lead to loss of recall at later time points. Disruption at 30 min blocks ITM and LTM recall at 3 and 4 h, respectively, whereas disruption at 2 h only blocks a late form of LTM at 24 h. Our results link transitions between phases of memory to both memory lapses and the susceptibility of memory to behavioural disturbance at specific time points after learning. Lapses in memory recall during consolidation in vitro Lapses in memory recall were first noticed in the in vitro associative conditioning experiments . In vitro conditioning of feeding using chemical stimuli is carried out in a semi-intact preparation ( Fig. 1a ) consisting of the retained sensory structures, the lips and oesophagus, connected by sensory nerves to the feeding circuits that are located in the buccal and cerebral ganglia [10] , [19] . Using a previously developed protocol [17] (see Methods) amyl acetate, the conditioned stimulus (CS) is paired with sucrose, the unconditioned stimulus (US) and response to the CS alone tested at various time points after a single CS+US pairing. Responses to the CS are recorded intracellularly as a sequence of bursts of spikes in identified feeding motoneurons such as the B4 ( Fig. 1a ) that is known to underlie feeding behaviour in the intact animal [12] . This pattern of electrical activity is termed ‘fictive feeding’ and is routinely used as a systems-level electrophysiological correlate of the behavioural conditioned response [16] , [20] . The fictive feeding pattern recorded in motoneurons requires the coordinated synaptic inputs from all the neurons of the feeding network including the feeding central pattern generator interneurons ( Fig. 1b ) [21] and modulatory interneurons [22] . It therefore represents the outcomes of changes due to learning in the whole-feeding network. 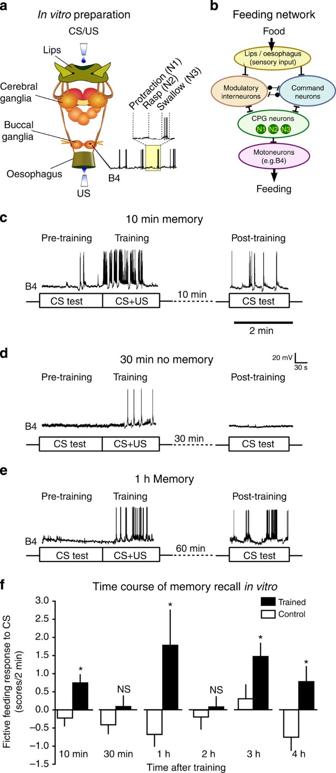Figure 1:Discontinuous expression of theinvitromemory. (a) Semi-intact preparation used forin vitroconditioning. (Details in Methods). Each cycle of feeding activity (expanded trace) in B4 can be divided into protraction (N1), rasp (N2) and swallow (N3) phases. The B4 fires during the swallow phase. (b) Summary of the feeding circuitry. Motoneurons such as the B4 are driven by cyclical synaptic inputs from three types of interneuron, N1, N2 and N3 that form the feeding central pattern generator (CPG). Food applied to the lips or oesophagus activates sensory input to command and modulatory interneurons that activate and control the CPG. (c) Example of a 10-min memory. The application of the CS post training is followed by bursts of fictive feeding activity in the B4 motoneuron. Also shown is the weaker pre-training response to the CS and the strong fictive feeding pattern induced by US application during CS+US pairing. (d) Example of memory lapse at 30 min. No spike activity is recorded in B4 in response to the CS at 30 min post training. (e) Example of the memory test 1 h after the training. There is strong fictive feeding response both during training and test as indicated by the strong bursting activity of the B4 cell. (f) Summary of time course and statistics. Memories were detected at 10 min, and 1, 3 and 4 h post training (two-tailed pairedt-test: 10 min group: df=18,P<0.01,N=19; 1 h group: df=20,P<0.003,N=21; 3 h group: df=18,P<0.005,N=19; 4 h group: df=14,P<0.02,N=15 for the) but not at 30 min and 2 h (pairedt-test: 30 min group: df=24,P>0.24,N=25; 2 h group: df =16,P>0.6,N=17). The negative pre-training scores (blank bars in Fig. 1f) result from the inhibition of background firing in feeding motoneurons by the CS before conditioning. The positive feeding scores following conditioning (dark bars in Fig. 1f) are not due to the reduction in this inhibitory effect but have previously been shown to involve the enhanced activation of excitatory pathways to the feeding network45. Asterisks indicate significance ofP<0.05. Errorbars show mean±s.e.m. Figure 1: Discontinuous expression of the in vitro memory . ( a ) Semi-intact preparation used for in vitro conditioning. (Details in Methods). Each cycle of feeding activity (expanded trace) in B4 can be divided into protraction (N1), rasp (N2) and swallow (N3) phases. The B4 fires during the swallow phase. ( b ) Summary of the feeding circuitry. Motoneurons such as the B4 are driven by cyclical synaptic inputs from three types of interneuron, N1, N2 and N3 that form the feeding central pattern generator (CPG). Food applied to the lips or oesophagus activates sensory input to command and modulatory interneurons that activate and control the CPG. ( c ) Example of a 10-min memory. The application of the CS post training is followed by bursts of fictive feeding activity in the B4 motoneuron. Also shown is the weaker pre-training response to the CS and the strong fictive feeding pattern induced by US application during CS+US pairing. ( d ) Example of memory lapse at 30 min. No spike activity is recorded in B4 in response to the CS at 30 min post training. ( e ) Example of the memory test 1 h after the training. There is strong fictive feeding response both during training and test as indicated by the strong bursting activity of the B4 cell. ( f ) Summary of time course and statistics. Memories were detected at 10 min, and 1, 3 and 4 h post training (two-tailed paired t -test: 10 min group: df=18, P <0.01, N =19; 1 h group: df=20, P <0.003, N =21; 3 h group: df=18, P <0.005, N =19; 4 h group: df=14, P <0.02, N =15 for the) but not at 30 min and 2 h (paired t -test: 30 min group: df=24, P> 0.24, N =25; 2 h group: df =16, P> 0.6, N =17). The negative pre-training scores (blank bars in Fig. 1f) result from the inhibition of background firing in feeding motoneurons by the CS before conditioning. The positive feeding scores following conditioning (dark bars in Fig. 1f) are not due to the reduction in this inhibitory effect but have previously been shown to involve the enhanced activation of excitatory pathways to the feeding network [45] . Asterisks indicate significance of P <0.05. Errorbars show mean±s.e.m. Full size image Examples of conditioned responses at 10 min ( Fig. 1c ) and 1 h ( Fig. 1e ) show that there is a significant increase in the fictive feeding response to the CS after conditioning compared with before training ( Fig. 1f ). The absence of a conditioned response (lapse in ‘memory’) at the 30 min time point is indicated by the lack of fictive feeding response to the CS after CS+US pairing ( Fig. 1d , statistics summarized in Fig. 1f legend). This is not due to the inability of the preparation to respond to chemical stimuli because both during training ( Fig. 1d ) and after training (data not shown) the US stimulated a feeding pattern. Similar results were obtained for a second lapse at 2 h ( Fig. 1f ). To examine whether the in vitro memory trace was specific to the association between the CS and the US, preparations that were exposed to US alone and CS alone were tested and compared with the paired ones. In these control groups the pairing of the CS+US was replaced by presentation of either the US for 2 min to both lips and oesophagus (US alone group) or by the presentation of the CS to the lips for 4 min (CS alone group). The semi-intact preparations were ideally suited for CS and US alone control tests as these stimuli can be applied at exactly the same time before the CS test as the CS and US pairing during the training. This would be impossible with unpaired controls as in that case an hour would be needed between the application of the two stimuli [1] . By using one-way ANOVAs (analysis of variance) we show that paired preparations responded significantly higher to the CS at 10 min (ANOVA F (2, 56) =7.3, P <0.01; Tukey’s tests: CS alone ( N =20) versus CS+US ( N =19), P <0.01; US alone ( N =20) versus CS+US, P <0.05; US alone versus CS alone, P >0.05 ), 1 h (F (2, 55) =5.2, P <0.01; Tukey’s tests: CS alone ( N =19) versus CS+US ( N =21), P <0.05; US alone ( N =19) versus CS+US, P <0.05; US alone versus CS alone, P >0.05 ), 3 h (ANOVA F (2, 48) =5.9, P <0.01; Tukey’s tests: CS alone ( N =17) versus CS+US ( N =17), P <0.01; US alone ( N =17) versus CS+US, P <0.05; US alone versus CS alone, P >0.05) and 4 h (ANOVA F (2, 38) =5.5, P <0.01; Tukey’s tests: CS alone ( N =13) versus CS+US ( N =15), P <0.05; US alone ( N =13) versus CS+US, P <0.05; US alone versus CS alone, P >0.05). Compiling the data from the in vitro experiments ( Fig. 1f ), shows memory lapses at 30 min and 2 h but not at 10 min, 1, 3 and 4 h after conditioning. Separate sets of experiments were performed for each time point to avoid repeated testing of the same preparation. Each preparation was tested before and after training and these feeding responses were compared ( Fig. 1f ). Lapses in recall during memory consolidation in vivo As the in vitro preparations have weakened sensory responses to food stimuli compared with the intact animal [20] , [23] , we reduced the concentration of the US in our one-trial behavioural conditioning experiments. Under these conditions, lapses in memory were revealed at the same time points, 30 min and 2 h that were detected in the in vitro experiments ( Fig. 2a ). Reducing the strength of the US (to 0.067% sucrose) was necessary to reveal these underlying weaknesses in memory recall because the higher US concentrations (0.67% sucrose) that were previously used for behavioural training produced a continuous, uninterrupted memory trace during consolidation with no lapses in memory ( Fig. 2b ). 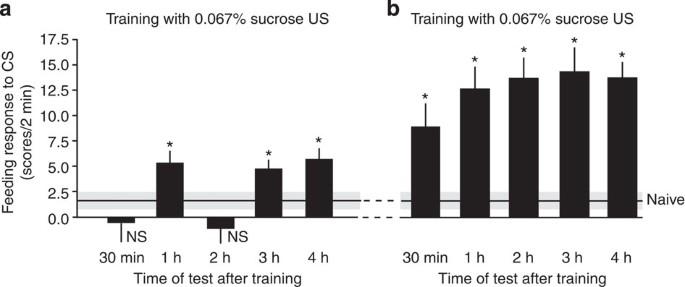Figure 2: Behavioural memory trace after one-trial conditioning. (a) Test of the conditioned response at 30 min, and 1, 2, 3, and 4 h after training with the low concentration of US (0.004% amyl acetate CS paired with 0.067% sucrose) resulted in significantly elevated responses only at the 1, 3 and 4 h time points compared with naïve, at all time points. Kruskal–Wallis statistics showed that there was a source of significant difference (H=29.26,P<0.0001) and Dunn’spost hoctest proved that the 30 min and 2 h groups were similar to naives (P<0.05 for 1, 3 and 4 hN=16–18,P>0.05 for the 30 min and 2 h groupsN=18 in each, naive:N=18). (b) Test of the conditioned response at 30 min, and 1, 2, 3, and 4 h after training with the high concentration of US (0.004% amyl acetate CS paired with 0.67% sucrose) resulted in significantly elevated responses compared with naïve, at all time points. Kruskal–Wallis statistics showed that there was a source of significant difference (H=26.88,P<0.0001) and Dunn’spost hoctest proved that all the groups tested at different time points scored significantly higher than the naïve control (*P<0.05 at each time point,N=17–20). Error bars show means+s.e.m. Figure 2: Behavioural memory trace after one-trial conditioning. ( a ) Test of the conditioned response at 30 min, and 1, 2, 3, and 4 h after training with the low concentration of US (0.004% amyl acetate CS paired with 0.067% sucrose) resulted in significantly elevated responses only at the 1, 3 and 4 h time points compared with naïve, at all time points. Kruskal–Wallis statistics showed that there was a source of significant difference ( H =29.26, P <0.0001) and Dunn’s post hoc test proved that the 30 min and 2 h groups were similar to naives ( P <0.05 for 1, 3 and 4 h N =16–18, P >0.05 for the 30 min and 2 h groups N =18 in each, naive: N =18). ( b ) Test of the conditioned response at 30 min, and 1, 2, 3, and 4 h after training with the high concentration of US (0.004% amyl acetate CS paired with 0.67% sucrose) resulted in significantly elevated responses compared with naïve, at all time points. Kruskal–Wallis statistics showed that there was a source of significant difference ( H =26.88, P <0.0001) and Dunn’s post hoc test proved that all the groups tested at different time points scored significantly higher than the naïve control (* P <0.05 at each time point, N =17–20). Error bars show means+s.e.m. Full size image Memory susceptibility coincides with memory phase transitions We hypothesized that the absence of conditioned responses at 30 min and 2 h occur at the transitions between different phases of memory. These phases are defined by their dependence on transcription and translation that occur early in the post-training period [24] , [25] , [26] , [27] , [28] . We used the translational blocker anisomycin (ANI) and the transcriptional blocker actinomycin-D (Act-D) to map out the three main phases of memory; STM, ITM and LTM using a mixture of in vitro and behavioural protocols that have previously been shown to be successful in Lymnaea [14] , [18] and are justified in the Methods section. We used the behavioural training procedure that is known to produce uninterrupted memory recall throughout the consolidation period. By using this protocol we aimed to reveal periods of susceptibility at times coinciding with the lapses observed after training with the weakened US or in vitro training. The 30 min lapse coincides with the transition from STM at 10 min to ITM at 1 h. The 10 min memory trace was shown to be a classic example of STM because it required neither de novo protein nor RNA synthesis. Neither ANI nor Act-D prevented the expression of the 10 min memory trace ( Fig. 3a ). The 1 h memory trace ( Fig. 3b ) has the accepted characteristics of ITM having a requirement for protein synthesis but no requirement for de novo mRNA synthesis [8] , [26] , [29] , [30] . Similar data were obtained for the 2 and 3 h memory traces using behavioural experiments for both types of blocker (unpaired t -test, 2 h Act-D: df=42, P >0.7; 2 h ANI: df=36, P <0.0001; 3 h Act-D: df=43, P >0.5; 3 h ANI: df=39, P <0.0001, Fig. 3c ). So the 1, 2 and 3 h memories are classified as ITM on the basis of their requirement for protein, but not RNA synthesis. As the second lapse of memory occurred at 2 h we asked whether this time point coincided with another transition between memory phases and their molecular dependencies. We therefore hypothesized that the 2 h lapse occurs at a transition between two types of ITM. Perhaps ITM has an early and a late phase, differing only in their requirements for specific protein kinases. To examine this possibility, we carried out experiments using protein kinase inhibitors to investigate the molecular requirement of the 2 h time point in more detail. First, we inhibited protein kinase A (PKA) using H-89, because it had previously been used successfully to block PKA activity after one-trial conditioning in Lymnaea [31] . All three time points tested (1, 2 and 3 h) were found to be PKA activity-dependent and so H-89 induced loss of memory recall Fig. 4 . 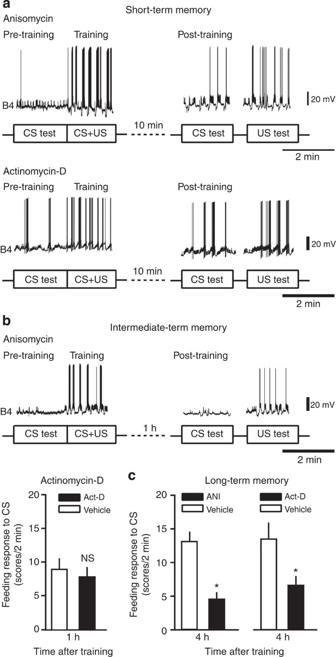Figure 3: Identification of different phases of memory. (a)The memory at 10 min is STM as characterized by the lack of requirement for protein and RNA synthesis. The post-training response of the B4 neuron to the CS at 10 min persists despite the presence of the protein synthesis inhibitor ANI (anisomycin) (pairedt-test; df=17,P<0.01,N=18). The memory is also unaffected by the RNA synthesis inhibitor Act-D (actinomycin-D) in other preparations (pairedt-test; df=18,P<0.01,N=10). (b) The memory at 1 h is ITM as characterized by the requirement for protein synthesis and the lack of requirement for new RNA synthesis. In the example shown here (btop trace) there was no difference in the pre-training B4 response to the CS prior compared with the CS response after training indicating that the conditioned response had been blocked by ANI. This is confirmed in the statistical analysis of the data from the whole group (pairedt-test; df=19,t=0.19,P>0.85,N=20). Act-D injected into intact animals did not affect the conditioned response 1 h after training. (vehicle-injected trained animals compared with Act-D injected trained animals, unpairedt-test; df=31,P>0.4,N=17). (c) The 4 h memory trace is LTM because it requires both protein and RNA synthesis. ANI and Act-D both blocked the memory trace compared with vehicle-injected controls (unpairedt-tests: ANI; df=42,P<0.0001; Act-D; df=42,P<0.0001). For earlier time points (up to 1 h), we usedin vitrotechniques, because injecting ANI into intact animals prevents normal feeding responses to sucrose and thus impairs acquisition18. Whole animal, behavioural experiments were used at later time points when the performance of the animals was not affected by the drugs’ side effects. All the training was done using the high US (0.67%) concentration. Asterisks indicate significance ofP<0.05. Error bars show means+s.e.m. Figure 3: Identification of different phases of memory. ( a )The memory at 10 min is STM as characterized by the lack of requirement for protein and RNA synthesis. The post-training response of the B4 neuron to the CS at 10 min persists despite the presence of the protein synthesis inhibitor ANI (anisomycin) (paired t -test; df=17, P <0.01, N =18). The memory is also unaffected by the RNA synthesis inhibitor Act-D (actinomycin-D) in other preparations (paired t -test; df=18, P <0.01, N =10). ( b ) The memory at 1 h is ITM as characterized by the requirement for protein synthesis and the lack of requirement for new RNA synthesis. In the example shown here ( b top trace) there was no difference in the pre-training B4 response to the CS prior compared with the CS response after training indicating that the conditioned response had been blocked by ANI. This is confirmed in the statistical analysis of the data from the whole group (paired t -test; df=19, t =0.19, P >0.85, N =20). Act-D injected into intact animals did not affect the conditioned response 1 h after training. (vehicle-injected trained animals compared with Act-D injected trained animals, unpaired t -test; df=31, P >0.4, N =17). ( c ) The 4 h memory trace is LTM because it requires both protein and RNA synthesis. ANI and Act-D both blocked the memory trace compared with vehicle-injected controls (unpaired t -tests: ANI; df=42, P <0.0001; Act-D; df=42, P <0.0001). For earlier time points (up to 1 h), we used in vitro techniques, because injecting ANI into intact animals prevents normal feeding responses to sucrose and thus impairs acquisition [18] . Whole animal, behavioural experiments were used at later time points when the performance of the animals was not affected by the drugs’ side effects. All the training was done using the high US (0.67%) concentration. Asterisks indicate significance of P <0.05. Error bars show means+s.e.m. 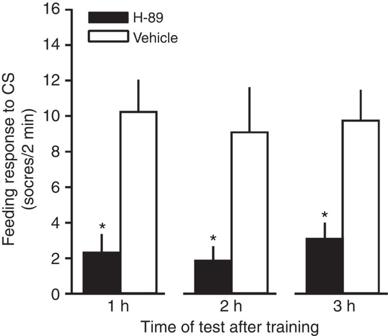Figure 4: Early PKA activation is required for both early and late ITM. Injection of the PKA inhibitor (H-89) immediately after training prevented memory expression when tested 1 h (H-89:N=18, vehicle:N=18) 2 h (H-89:N=18, vehicle:N=18) and 3 h (H-89:N=18, vehicleN=18) after training. Statistical analysis (un-pairedt-tests) showed that there was a significant difference between the drug and the vehicle-injected groups at each time point tested (1 h:P<0.001, 2 h:P<0.008, 3 h:P<0.004). A one-way ANOVA test of all the drug-injected groups showed no difference between the three groups (P>0.7) and the same analysis also proved that the vehicle-injected groups performed similarly at the memory tests at each time points (P>0.9). Asterisks indicate significance ofP<0.05. Error bars show means+s.e.m. Full size image Figure 4: Early PKA activation is required for both early and late ITM. Injection of the PKA inhibitor (H-89) immediately after training prevented memory expression when tested 1 h (H-89: N =18, vehicle: N =18) 2 h (H-89: N =18, vehicle: N =18) and 3 h (H-89: N =18, vehicle N =18) after training. Statistical analysis (un-paired t -tests) showed that there was a significant difference between the drug and the vehicle-injected groups at each time point tested (1 h: P <0.001, 2 h: P <0.008, 3 h: P <0.004). A one-way ANOVA test of all the drug-injected groups showed no difference between the three groups ( P >0.7) and the same analysis also proved that the vehicle-injected groups performed similarly at the memory tests at each time points ( P >0.9). Asterisks indicate significance of P <0.05. Error bars show means+s.e.m. Full size image Second, we injected the protein kinase C (PKC) blocker, bisindolylmaleimide-1 (Bis), immediately after training and tested for memory recall at the same time points as before. At the 10 μM concentration we used Bis is specific for PKC [32] . Injected animals were amnesic at 1 h and 2 h but not at 3 h ( Fig. 5a ), suggesting that PKC is not required for a late phase of ITM. However, a constitutive variant of PKC, protein kinase M (PKM), could be required for the second phase of ITM so we injected the PKM inhibitor, 5 μM chelerythrine immediately after training. Chelerythrine at this low concentration is known to specifically inhibit atypical members of the PKC family, including PKM [32] . We found that memory at 1, 2 and 3 h was PKM-dependent ( Fig. 5b ). These results show that there are differences in the molecular dependencies of an early (1 and 2 h) and a late phase (3 h) of ITM. Early ITM requires both PKC and PKM while late ITM only requires PKM. These findings suggest that the lapse in memory recall at 2 h is due to a transition from PKC/PKM-dependent phase of ITM to a PKM-dependent phase of ITM. LTM at 4 and 24 h is neither PKC ( Fig. 5a ) nor PKM-dependent ( Fig. 5b ) suggesting that the memory traces for ITM and LTM develop by using parallel pathways. 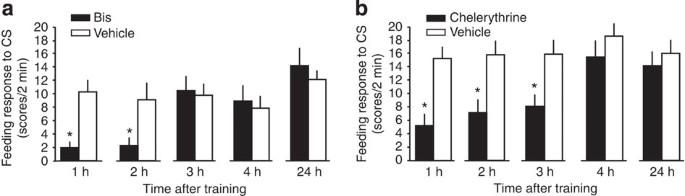Figure 5: Differential roles for PKC and PKM in the induction of early and late intermediate memory and long-term memory. (a) Injection of the PKC inhibitor Bis after training blocked the 1 and 2 h but not the 3 h or later memory trace, induced by training with the 0.67% US protocol, when compared with the vehicle-injected trained groups (unpairedt-tests, 1 h:P<0.0003 df=34, Bis:N=18, vehicle:N=18, 2 h:P<0.004, df=33, Bis:N=17, vehicle:N=18, 3 h:P>0.5, df=32, Bis:N=16, vehicle:N=18, 4 h:P>0.5, df=24, Bis:N=15, vehicle:N=18, 24 h:P>0.5, df=25, Bis:N=18, vehicle:N=18). (b) Injection of chelerythrine (CH) after training (5 μM final concentration) blocked the memory up to 3 h after training. With the high US concentration but from 3 h the memory becomes independent of PKM. (Unpairedt-tests, 1 h:P<0.0007 df=33, CH:N=18, vehicle:N=18, 2 h:P<0.004, df=33, CH:N=18, vehicle:N=18, 3 h:P<0.005, df=33, CH:N=18, vehicle:N=18, 4 h:P>0.5, df=33, CH:N=18, vehicle:N=18, 24 h:P>0.5, df=33, CH:N=18, vehicle:N=18). Asterisks indicate significance ofP<0.05. Error bars show means+s.e.m. Figure 5: Differential roles for PKC and PKM in the induction of early and late intermediate memory and long-term memory. ( a ) Injection of the PKC inhibitor Bis after training blocked the 1 and 2 h but not the 3 h or later memory trace, induced by training with the 0.67% US protocol, when compared with the vehicle-injected trained groups (unpaired t -tests, 1 h: P <0.0003 df=34, Bis: N =18, vehicle: N =18, 2 h: P <0.004, df=33, Bis: N =17, vehicle: N =18, 3 h: P >0.5, df=32, Bis: N =16, vehicle: N =18, 4 h: P >0.5, df=24, Bis: N =15, vehicle: N =18, 24 h: P >0.5, df=25, Bis: N =18, vehicle: N =18). ( b ) Injection of chelerythrine (CH) after training (5 μM final concentration) blocked the memory up to 3 h after training. With the high US concentration but from 3 h the memory becomes independent of PKM. (Unpaired t -tests, 1 h: P <0.0007 df=33, CH: N =18, vehicle: N =18, 2 h: P <0.004, df=33, CH: N =18, vehicle: N =18, 3 h: P <0.005, df=33, CH: N =18, vehicle: N =18, 4 h: P >0.5, df=33, CH: N =18, vehicle: N =18, 24 h: P >0.5, df=33, CH: N =18, vehicle: N =18). Asterisks indicate significance of P <0.05. Error bars show means+s.e.m. Full size image No lapses in memory in either the in vitro conditioning experiments ( Fig. 1f ) or the in vivo experiments ( Fig. 2a ) occurred between 3 and 4 h, even though this is a transition period between ITM and LTM. At this transition there is a change from RNA synthesis independence (ITM) to RNA synthesis dependence (LTM). Four hours is the first time point at which expression of the memory trace requires both protein and RNA synthesis ( Fig. 3c ). Thus, it appears that the rule that transitions in molecular mechanisms coincide with lapses in memory does not apply once late ITM progresses into LTM because new proteins required for LTM were synthesized at an earlier stage. All the above experiments were performed by using the training paradigm with the high sucrose (US) concentration. However, training with the low sucrose (US) concentration, which reveals lapses in vivo at 30 min and 2 h, may in principle use molecular processes different from those activated by high sucrose training. To examine this possibility we tested whether training with low sucrose also leads to protein synthesis-dependent ITM at 3 h and RNA and protein synthesis-dependent LTM at 4 and 24 h. Act-D or ANI or the vehicle solution was injected immediately after training with the reduced US concentration into three groups of snails. Separate groups of randomly chosen animals were tested at 3, 4 and 24 h after training and the drug-injected groups were compared with trained animals injected with vehicle solution ( Fig. 6 ). The results show that, as was the case with the high US concentration training, conditioning with the low concentration sucrose also leads to translation-dependent ITM at 3 h and transcription and translation-dependent LTM at 4 and 24 h after training. 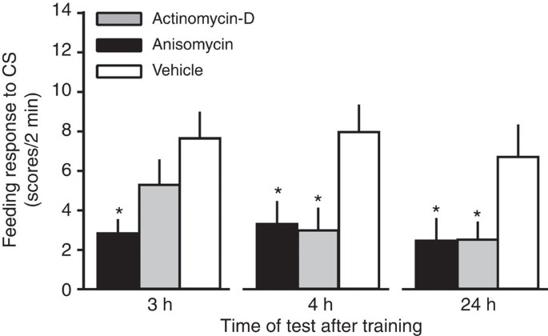Figure 6: Identification of memory phases after training with the low US concentration. Just as was the case with the high US concentration, the memory at 3 h is also considered to be ITM as characterized by the requirement for protein synthesis and the lack of requirement for new RNA synthesis. Statistical analysis of the 3 h data showed that there was significant difference among the groups (one-way ANOVAP<0.05) and the source of this difference was between the ANI and the vehicle-injected groups (Dunn’spost hoctestP<0.05) while there was no statistical difference between the Act-D and the vehicle-injected groups (P>0.05) (ANI:N=16, Act-D:N=16 vehicle:N=18). The same tests showed that at 4 and 24 h the memory trace can be classified as LTM. The responses in both of the drug-injected groups were significantly reduced compared with the vehicle-injected ones (one-way ANOVAP<0.05 for both, 4 h: ANI:N=17, Act-D:N=18, vehicle:N=17, 24 h: ANI:N=18, Act-D:N=18, vehicle:N=17). Asterisks indicate significance ofP<0.05. Error bars show means+s.e.m. Figure 6: Identification of memory phases after training with the low US concentration. Just as was the case with the high US concentration, the memory at 3 h is also considered to be ITM as characterized by the requirement for protein synthesis and the lack of requirement for new RNA synthesis. Statistical analysis of the 3 h data showed that there was significant difference among the groups (one-way ANOVA P <0.05) and the source of this difference was between the ANI and the vehicle-injected groups (Dunn’s post hoc test P <0.05) while there was no statistical difference between the Act-D and the vehicle-injected groups ( P >0.05) (ANI: N =16, Act-D: N =16 vehicle: N =18). The same tests showed that at 4 and 24 h the memory trace can be classified as LTM. The responses in both of the drug-injected groups were significantly reduced compared with the vehicle-injected ones (one-way ANOVA P <0.05 for both, 4 h: ANI: N =17, Act-D: N =18, vehicle: N =17, 24 h: ANI: N =18, Act-D: N =18, vehicle: N =17). Asterisks indicate significance of P <0.05. Error bars show means+s.e.m. Full size image Susceptibility of memory expression in consolidation We propose that associative memory consolidation might become susceptible to interference at specific times. To test this hypothesis, we disturbed the animals using a novel mechanical stimulus at 10 and 30 min, and 1 and 2 h after training and tested for recall at 3, 4 and 24 h after training. A mildly aversive mechanical stimulus was applied to the foot sufficient to evoke a local retraction. We used the behavioural training procedure that is known in undisturbed animals to produce an uninterrupted memory throughout the consolidation period. By using this protocol, we aimed to reveal periods of susceptibility at times coinciding with the lapses observed after training with the low sucrose US or in vitro training. As before, separate groups of animals were tested for recall at each time point. Disturbance at 30 min and 2 h, but not at 10 min and 1 h, blocked recall at later time points ( Fig. 7 ). The mechanical stimulus applied at 30 min after training blocked memory recall at 3 ( Fig. 7a ) and 4 h ( Fig. 7b ) compared with the undisturbed trained group (labelled control in Fig. 7a–c ) tested at the same times. 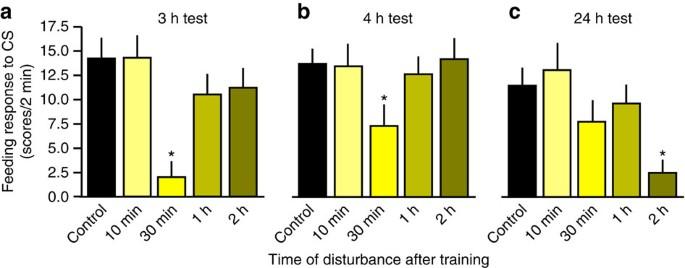Figure 7: Disruption of the memory at 30 min and 2 h results in loss of memory expression at later time points. Separate groups of animals were disturbed at 10 and 30 min, 1 and 2 h after training by applying a mechanical stimulus to the foot. There was another group of animals which only received the training but was not exposed to any disturbance. Randomly selected animals (N=16–18 for each testing time) from all the groups were tested at 3, 4 and 24 h after the training. Data were analysed by using Kruskal–Wallis tests followed by Dunn’spost hoctest for each testing time. Kruskal–Wallis statistics showed that there was a source of significant difference at all testing times (3 h:H=16.35,P<0.003; 4 h:H=8.4,P<0.04; 24 h:H=13.9,P<0.007). With thepost hocanalysis of all treated groups were compared with the trained undisturbed control group (black bars). At the 3 h testing time (a) only the group that received the disturbance 30 min after training was significantly different from the control (H=16.35,P<0.003). At the 4 h testing time (b) again only the group disturbed at 30 min was different from the control (H=8.4,P<0.04). At the 24 h test (c) only the group that was disturbed 2 h after training was different from the controls (H=13.9,P<0.007). Asterisks indicate significance ofP<0.05. Error bars show means+s.e.m. Figure 7: Disruption of the memory at 30 min and 2 h results in loss of memory expression at later time points. Separate groups of animals were disturbed at 10 and 30 min, 1 and 2 h after training by applying a mechanical stimulus to the foot. There was another group of animals which only received the training but was not exposed to any disturbance. Randomly selected animals ( N =16–18 for each testing time) from all the groups were tested at 3, 4 and 24 h after the training. Data were analysed by using Kruskal–Wallis tests followed by Dunn’s post hoc test for each testing time. Kruskal–Wallis statistics showed that there was a source of significant difference at all testing times (3 h: H =16.35, P <0.003; 4 h: H =8.4, P <0.04; 24 h: H =13.9, P <0.007). With the post hoc analysis of all treated groups were compared with the trained undisturbed control group (black bars). At the 3 h testing time ( a ) only the group that received the disturbance 30 min after training was significantly different from the control ( H =16.35, P <0.003). At the 4 h testing time ( b ) again only the group disturbed at 30 min was different from the control ( H =8.4, P <0.04). At the 24 h test ( c ) only the group that was disturbed 2 h after training was different from the controls ( H =13.9, P <0.007). Asterisks indicate significance of P <0.05. Error bars show means+s.e.m. Full size image Disturbance at 2 h caused recall loss at 24 h ( Fig. 7c ) but not at 3 ( Fig. 7a ) or 4 h ( Fig. 7b ). Disturbances at 10 min and 1 h had no effect on later memory recall compared with trained controls at all three test points (3 h, Fig. 7a ; 4 h, Fig. 7b ; 24 h, Fig. 7c ). Post hoc tests proved that at the 3 and 4 h tests only the groups that were disturbed 30 min after the training showed significantly reduced response to the CS compared with controls while at 24 h it was the group disturbed 2 h after the training that scored significantly lower than controls (detailed statistics in legends to Fig. 7 ). These results show that susceptibility is only present when the external disturbance coincides with the two lapses in memory revealed above. Our previous result on one-trial chemical conditioning of feeding behaviour in Lymnaea [16] suggested that memory consolidation is a continuous process. However, using an in vitro conditioning paradigm and a modified version of behavioural conditioning here we show that the structure of consolidation is more complex. Periods of susceptibility of memory consolidation are indicated by brief lapses in memory that occur at specific time points following conditioning. Significantly, both methods of assaying memory recall revealed lapses in memory at the same time points, 30 min and 2 h after training. We show here that the two lapses observed in our experiments coincide with the periods when there is a change in molecular mechanisms only at the early stages of memory formation. So it seems that recall of memory becomes more difficult when there are changes in molecular dependencies indicating that distinct molecular pathways are responsible for the different phases of memory formation [33] , [34] . Our previous experiments revealed that these essential changes in molecular requirements are initiated following a single training trial during an early stage of memory consolidation [18] , [35] . Subsequent downstream mechanisms cause recall between STM and early ITM (at 30 min) and between early and late ITM (at 2 h) to become inherently weaker and susceptible. We used the training paradigm leading to uninterrupted memory to test for mechanisms of recall failure at the critical times in our pharmacological blocking experiments. This raised the question whether the two training paradigms result in memories using similar or distinct molecular processes. Our results show that both training paradigms induced the same translation but not transcription- dependent ITM at 3 h and protein and RNA synthesis-dependent LTM at 4 and 24 h. During STM covalent modification of existing proteins can lead to changes in properties of ion channels resulting in increased excitability or enhance synaptic transmission. This process lasts for at least 10 min after training. Between the 10 min and 1 h time period there is a transition to translation-dependent ITM that lasts up to 3 h after training. During this period newly synthesized proteins from existing RNA can contribute to enhance efficacy of synapses for example by the insertion of more channel proteins into the cell membrane at the active zone. ITM is thought to be dependent on downstream processes, such as activation of silent presynaptic terminals by translationally dependent but transcriptionally independent filling of pre-existing empty varicosities with synaptic vesicles, which lasts for several hours. During the early period of ITM intracellular cascades induced by PKC activation can lead to for example, mobilization of vesicles or simultaneous pre- and post-synaptic modifications, like in intermediate-term facilitation in Aplysia [36] , [37] . The late phase of ITM differs from the early one in its independence of PKC but dependence on PKM-induced processes. LTM may involve both the modification of existing synapses and the construction of new synapses that requires both transcription and translation [26] , [36] , [38] . New synapses continue to be produced for up to at least 24 h and this is consistent with LTM in Lymnaea, which can be recorded for 24 h and beyond [16] . We showed that both the 4 and 24 h LTM were PKC and PKM independent. Early and late LTM, however, differ in their requirement for the duration of PKA activity following training [31] . 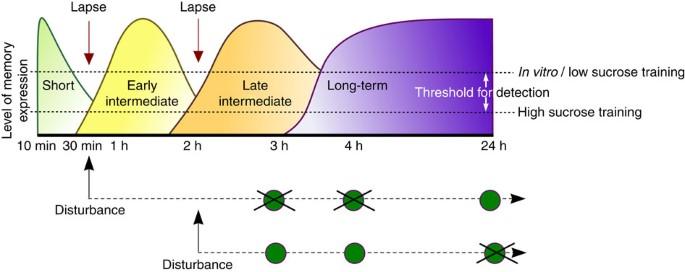Figure 8: Schematic representation of the time course of four phases of memory following associative conditioning. Time since conditioning is plotted against the hypothetical level of memory expression. Each curve represents a different form of memory (short-term, early intermediate, late intermediate and long-term). The two dashed lines indicate the read-out (threshold) of the memory trace after training with the high (0.67%) and the low (0.067%) concentrations of sucrose (US). The lower threshold for the conditioning with the high US concentration leads to the detection of memory at all time points. The higher threshold for training with the low US concentration orin vitroaccounts for the lapse in the memory at 30 min and 2 h at transitions between short- and early ITM and early and late ITM, respectively (red arrows). Semi-intact preparations tend to have lower levels of response to sensory stimuli than whole animals inLymnaea20,23and in other molluscs (for example,Limax)46and this accounts for the higher detection threshold forin vitromemory expression. The absence of a lapse in memory between 3 and 4 h is because the expression level of the memory trace is above the threshold for memory recall. Upward arrows indicate the time points when the mechanical disturbance was applied and the behavioural effect on subsequent phases of memory indicated by the green spots. Crossed green spots indicate failure of recall. Disturbance was applied at other time points but had no effect (omitted for clarity). Figure 8 shows a schematic diagram of the time course of the four phases of memory. The model assumes that the level of memory expression rises and falls during each of the initial phases of memory consolidation, before becoming stabilised when the memory enters the long-term phase. Also incorporated in the model is the proposal that the type of training alters the threshold (dashed lines) at which the memory can be detected either behaviourally in vivo or fictively in vitro . Thus, this simple informal model accounts for the lapses of the memory at phase transitions during consolidation. It also accounts for the continuous memory expression (no lapses during consolidation) that occurs following behavioural training with high US concentration. The model assumes that the molecular mechanisms leading to lapses in memory in vitro are present in the high sucrose experiments but do not express themselves as lapses of memory recall because of the lower threshold for detection of the memory trace. We cannot be absolutely certain of this but it is supported by earlier experiments when comparisons of data obtained in vitro and in vivo from the same one-trial high-sucrose training showed similar nitric oxide and protein synthesis dependence for different phases of memory consolidation [13] , [14] , [18] . There is a general acceptance in the molluscan learning literature that molecular mechanisms for in vitro and behavioural conditioning are directly comparable [39] . Figure 8: Schematic representation of the time course of four phases of memory following associative conditioning. Time since conditioning is plotted against the hypothetical level of memory expression. Each curve represents a different form of memory (short-term, early intermediate, late intermediate and long-term). The two dashed lines indicate the read-out (threshold) of the memory trace after training with the high (0.67%) and the low (0.067%) concentrations of sucrose (US). The lower threshold for the conditioning with the high US concentration leads to the detection of memory at all time points. The higher threshold for training with the low US concentration or in vitro accounts for the lapse in the memory at 30 min and 2 h at transitions between short- and early ITM and early and late ITM, respectively (red arrows). Semi-intact preparations tend to have lower levels of response to sensory stimuli than whole animals in Lymnaea [20] , [23] and in other molluscs (for example, Limax ) [46] and this accounts for the higher detection threshold for in vitro memory expression. The absence of a lapse in memory between 3 and 4 h is because the expression level of the memory trace is above the threshold for memory recall. Upward arrows indicate the time points when the mechanical disturbance was applied and the behavioural effect on subsequent phases of memory indicated by the green spots. Crossed green spots indicate failure of recall. Disturbance was applied at other time points but had no effect (omitted for clarity). Full size image An important finding of the present paper is that the transitions between phases, when the memory recall is at its weakest, are key points when the process of consolidation is susceptible to novel external stimuli. These lapses seem to reflect an inbuilt mechanism of susceptibility because application of a mildly aversive external stimuli still interfere with LTM formation, even when optimal training would otherwise have produced continuous memory trace with no overt lapses. The sensitivity of the mechanism of consolidation at transitions suggests the existence of choice points or ‘gates’ when the ‘automatic’ progression through to LTM can be prevented. The mildly aversive stimulus used in the disturbance experiment, leads to a local withdrawal response, a behaviour which is known to take precedence over feeding in a hierarchy of behavioural organization [40] . We show that this can prevent the subsequent conditioned feeding behaviour in the long-term. There is an early (4 h) and late (24 h) form of LTM [31] that are differentially blocked depending on which choice point is ‘disturbed’. Interestingly, disturbance at 30 min blocks recall at 4 h after training while the same stimulation at 2 h only affects the 24 h memory. This also indicates that there are independent, parallel pathways acting during memory formation. More generally, we speculate that the choice points our experiments have revealed allow memory to be expressed adaptively according to a variety of internal (for example, hunger and satiety [41] ), and external stimuli or variation in the strength of associations between different environmental stimuli [42] , [43] . Periods of recall susceptibility could therefore provide opportunities for novel external stimuli to alter the fate of a consolidating memory trace. Animals All the experiments were carried out on adult pond snails, Lymnaea stagnalis , aged between 4 and 6 months and raised in our laboratory. The animals were kept in copper-free water at 19–22 °C, with a 12 h light/12 h dark regime. They were fed three times a week with lettuce and twice a week with vegetable fish food (Tetra-Phyll; TETRA Werke, Melle, Germany). In vitro preparation and electrophysiological procedures The semi-intact preparation used for in vitro conditioning consisted of the entire CNS and chemo- sensory structures (that is, lips and oesophagus, Fig. 1a ). The preparations were perfused with normal saline (NS) containing 50 mM NaCl, 1.6 mM KCl, 2 mM MgCl2, 3.5 mM CaCl2, 10 mM HEPES buffer in water [44] . Intracellular recordings were made by using sharp electrodes (20–40 MΩ) filled with 4 M potassium acetate. NL 102 (Digitimer Ltd) and Axoclamp 2A (Axon Instrument, Molecular Device) amplifiers were used and data were acquired using a micro 1401 Mk II interface and analysed using Spike 2 software (Cambridge Electronic Design, Cambridge, UK). The semi-intact preparations were conditioned by perfusing the lips with 0.004% amyl acetate (CS) in NS for 2 min, immediately followed by 2 min of 0.004% amyl acetate applied to the lips together with 0.67% sucrose (US) perfused both to the lips and oesophagus. The conditioned response was tested by perfusing the lips with the CS for 2 min and measuring the electrophysiological response in the B1, B3, B4 feeding motoneurons recorded at various time points (10 and 30 min, 1, 2, 3 and 4 h) in separate experiments, after the one-trial conditioning. These motoneurons were selected to measure fictive feeding in response to the CS because they easily can be identified due to their large size and established location on the surface of the buccal ganglia [19] . Fictive feeding consists of a series of bursts of spikes corresponding to feeding cycles in the intact animal [21] . Fictive feeding responses were measured as the frequency of feeding bursts in the 2 min after application of the CS ( Fig. 1 ). Spontaneous rates of fictive feeding were also measured in the 2 min period before application of the CS for comparison. The US was perfused for 2 min to the lips beginning 5 min after the end of the CS test to check that the normal chemosensory pathways were intact and functional in the preparation. The preparations showing no fictive feeding response to the US either during pairing or at the subsequent US test were not analysed as part of the results. In vivo training procedure One-trial reward classical conditioning was performed by pairing amyl acetate, the CS with sucrose, the US using a previously well described method [17] , [41] . In one training protocol the sucrose US was applied at 0.67% concentration producing optimal robust learning, while in the other the CS was paired with a weaker US (0.067%) leading to a sub-optimal conditioning. In both protocols the CS concentration remained the same at 0.004%. After 2 days starvation animals were placed individually in petri dishes containing 90 ml copper-free water and left there to acclimatize for 10 min before each training procedure. Five millilitre of the amyl acetate solution (CS) was added to the water (0.004% final concentration) and 15 s later 5 ml of the US was applied. Animals were left in the solution containing the CS and the US for 2 min then rinsed and returned to their home tanks. In the drug experiments separate groups were injected with 100 μl of either the drug or the vehicle solution. To avoid interference with recall processes, separate groups of animals were trained for each time point and tested after training. It was necessary to use a combination of in vivo and in vitro techniques. On one hand, only the in vivo experiments allowed us to test the effect of drugs on memory at 2 h post training when the in vitro trace showed a lapse. On the other hand, testing drug effects on memory shortly after training in vivo is not possible because it requires the settling of animals in the test dish, which takes at least 10 min [43] . There are also side effects from ANI injection, not present in the in vitro preparations, that prevent normal feeding responses for up to 90 min after injection. For these reasons, the effect of ANI on memory at 10 min and 1 h post training could only be tested using the in vitro training protocol. Drug application All drugs were obtained from Sigma-Aldrich unless stated otherwise and were administered by injecting 100 μl of the drug solution into the haemolymph through the foot of the animals by using a fine syringe needle (gauge 30G ½, Sigma No: 305106). The absence of a blood–brain barrier allows the drugs free access to the central nervous system. The haemolymph volume is about 1 ml therefore the injected concentrations were calculated to be ten times the final concentrations. ANI and Act-D were applied in 10 μM final concentration diluted in 0.1% DMSO in saline. In the in vitro experiments ANI was perfused continuously throughout the pre- training and post-training periods. Under these conditions ANI is known to block protein synthesis in the Lymnaea CNS [18] but does not block the normal feeding response to sucrose in the semi-intact preparation ( Fig. 3ai , US test). 10 μM Act-D is known irreversibly to block RNA synthesis in the CNS after 1 h (ref. 18 ) so it was applied to the semi-intact preparation for 1 h before CS+US pairing in a separate group of preparations. Again Act-D does not prevent normal responses to sucrose ( Fig. 3aii ). Bisindolylmaleimide (Bis) (Calbiochem) (in 100% DMSO) was diluted with NS to achieve a 10 μM final concentration plus 0.1% DMSO. Chelerythrine was applied in 5 μM final concentration diluted in saline solution containing 0.1% DMSO. The PKA inhibitor H-89 was applied in 5 μM final concentration dissolved in NS with 0.1% DMSO. Data analysis The effects of conditioning on the CS response in both behavioural and in vitro electrophysiological experiments were assessed using ‘difference scores’. Difference scores were obtained by subtracting the number of feeding (behaviour) or fictive feeding cycles (electrophysiology) observed during water application in the behavioural experiments or in the 2 min preceding the CS application in the in vitro experiments from the number of cycles observed during CS application. The ‘blind’ analysis of the intracellular recording data was performed using Spike2 software (Cambridge Electronic Design, Cambridge, UK). The comparisons between groups have been carried out using two-tailed t -tests, paired t -tests were used when the same animals were tested repeatedly, unpaired t -test were used when two distinct groups of animals were compared. Multiple groups were tested by using analysis of the variance (one-way ANOVA) followed by a suitable post hoc test. The Kolmogorov–Smirnov (K–S) test was performed to decide on the use of either parametric or non-parametric test. The data collected from several experiments were analysed using the statistical software SPSS (SPSS Inc.) and GraphPad Prism (GraphPad Software Inc. San Diego, CA, USA). The K–S test showed that the normal distribution is an accurate approximation for the data sets collected from both behavioural and electrophysiological experiments. In addition to the K–S test the density function was plotted using the statistical software R (R-project) showing Gaussian distribution. In the in vitro conditioning experiments the minimum size of the sample required was calculated to be 16 with a power of at least 0.9 using the statistical software G*Power (Franz Faul, Universität Kiel, Germany). Cohen’s size effect was calculated from the earliest in vitro conditioning experiments ( d =0.8). In order to assess whether the CS had any effect before conditioning, naive responses to CS (difference scores) from each group were analysed. A one sample t -test against a hypothetical population with mean 0 showed no significant difference ( P <0.05, data not shown) for the populations analysed consistently with previous work from Straub et al . [45] How to cite this article: Marra, V. et al . Susceptibility of memory consolidation during lapses in recall. Nat. Commun. 4:1578 doi: 10.1038/ncomms2591 (2013).